A plasmid-based multigene expression system for mammalian cells The introduction of heterologous genetic information, particularly of multiple genes, into mammalian cells is a key technology in contemporary experimental biological research. The coexpression of fluorescently tagged sensors is required to simultaneously analyse multiple parameters in living cells and the coexpression of several proteins is necessary to manipulate cell fate in stem cell biology. Current technologies for multigene expression in mammalian cells are inefficient, inflexible and time-consuming. In this paper we describe MultiLabel, a novel and highly efficient modular plasmid-based eukaryotic expression system. Independent expression vectors are assembled by a Cre/ LoxP reaction into a plasmid with multiple expression cassettes. MultiLabel enables rapid construction of multigene expression vectors for the single-step creation of transiently or stably transfected mammalian cells. Genetic engineering of mammalian cells with multiple transgenes is an essential need in contemporary cell biology. Examples include the reprogramming of somatic cells into stem cells by coexpression of Oct3/4, Sox2, c-Myc and Klf4, or the simultaneous monitoring of multiple parameters in living cells with several fluorescent-protein-based sensors in cell biological studies [1] , [2] . Currently, this is achieved by sequential transfection of cells with plasmids, by co-transfection of several plasmids, by transfection with IRES-based polycistronic constructs, by the (self-)cleavage of larger precursor fusion proteins or by coinfection with several viruses such as Lentivirus vectors, each carrying a specific gene [3] , [4] , [5] . These approaches share in common one or more of the following disadvantages: there is a limited number of selection markers available for specific selection of transfected cells; restriction fragment-based cloning is cumbersome and standardization is difficult; the expression levels of individual proteins are not controllable; the delivery of unnecessary viral genes may alter the biological context of transfected cells; the cleavage from larger precursor proteins leads to proteins with modified N and C termini, which may compromise their function; the use of viruses requires special laboratory safety equipment; and, most importantly, it is virtually impossible to generate cell populations in which every cell simultaneously expresses all desired proteins. Our MultiLabel technology, in contrast, overcomes these impediments by using a single multigene plasmid that contains all genes of interest for transformation. For construction of this multigene plasmid, we adopted a Cre/ LoxP fusion-based donor–acceptor strategy that we had designed and successfully used previously for protein production in E. coli or insect cells for structural biology applications [6] , [7] . Briefly, an array of donor plasmids, each with a conditional origin of replication (from R6Kγ phage), is fused by an in vitro Cre/ LoxP reaction to an acceptor plasmid containing a common origin of replication (ColE1) [8] . The reaction mixture is then transformed into DH10β (pir-) bacteria and selected with appropriate antibiotics. Only fused plasmids can propagate because unfused donor plasmids with a conditional R6Kγ origin cannot replicate in DH10β cells. Desired donor–acceptor multigene fusions are then identified and selected in a process that can be automated [6] . Donors and acceptors contain the genes of interest, optionally tagged with a fluorescent marker and/or purification, immunolabelling or precipitation tag. We demonstrate that our MultiLabel system can be used for highly efficient transient coexpression of currently up to five genes of interest in transfected cells. In addition, MultiLabel enables the generation of stable multigene expresser cell lines, as the constructs carry the necessary antibiotic resistance selection markers and a unique homing endonuclease restriction site for linearization of the multigene plasmid. In this study, we show that it is possible to assemble several expression cassettes in a single plasmid in a modular way. Transiently transfected mammalian cells homogenously express all proteins and it is possible to generate stable cell lines expressing multiple transgenes in a single step. The viability of transfected cells is not affected as they show, for instance, the expected behaviour after stimulation with growth factors. We conclude that MultiLabel is a valuable tool for modifying mammalian cells with multiple genes. Vector design We have created a collection of DNAs representing regulatory elements that are combined to donor and acceptor plasmids. The size of these DNA elements was minimized to optimize transfection efficiency. Selectable markers for the generation of stable cell lines were introduced, and the junctions between the regulatory elements were standardized for optional high-throughput cloning and efficient reuse of existing expression cassettes. The construction of a multigene expression plasmid consists of only three simple steps ( Fig. 1 ). First, eight fragments were assembled in a single step to an acceptor or donor plasmid. This step is only required when an expression vector with entirely new features (for example, a new promoter or tag) is being built. A detailed overview of the construction, as well as the currently available vectors, is given in Supplementary Figures S1 , S2 and S3 . Second, the gene of interest was inserted by a cloning method of choice into the acceptor or donor, leading to an expression vector for a single protein. Existing expression cassettes from pcDNA- or pEGFP-based vectors can be easily transferred by PCR with standardized primers ( Supplementary Fig. S4 ). Finally, Cre-mediated recombination was used in vitro to assemble donor and acceptor vectors into a multiexpression plasmid, followed by transformation into E. coli and selection with an appropriate combination of antibiotics. Currently, we created eight donor vectors with four independent antibiotic resistance genes. They can be fused with one acceptor vector yielding a plasmid with up to five expression cassettes ( Supplementary Fig. S5 ). This plasmid array can be easily extended ad lib by introducing further antibiotic resistance markers. Additional expression cassettes can be inserted into each donor vector using a unique I-CeuI homing-endonuclease site in the special region ( Supplementary Fig. S6 ). 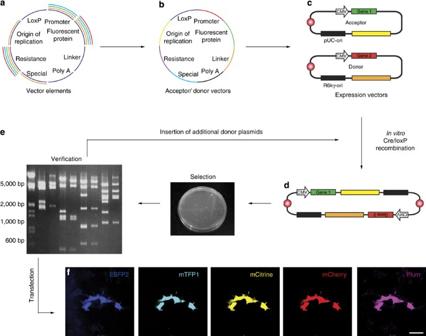Figure 1: Generation of a multiexpression plasmid. (a) A library of compatible regulatory elements was generated. Multiple lines for a fragment indicate available variations. (b) Donor and acceptor plasmids are created from this collection of regulatory elements. (c) The genes of interest are inserted into a donor or acceptor vector, leading to expression vectors for the desired genes. (d) One to four donor vectors are fused to one acceptor vector in a single step or in an iterative process. (e) Plasmids are selected by appropriate antibiotics and verified by restriction digestion. (f) Plasmids are then used to transfect mammalian cells. Scale bar, 50 μm. Figure 1: Generation of a multiexpression plasmid. ( a ) A library of compatible regulatory elements was generated. Multiple lines for a fragment indicate available variations. ( b ) Donor and acceptor plasmids are created from this collection of regulatory elements. ( c ) The genes of interest are inserted into a donor or acceptor vector, leading to expression vectors for the desired genes. ( d ) One to four donor vectors are fused to one acceptor vector in a single step or in an iterative process. ( e ) Plasmids are selected by appropriate antibiotics and verified by restriction digestion. ( f ) Plasmids are then used to transfect mammalian cells. Scale bar, 50 μm. Full size image Homogenous expression of five proteins from a single plasmid To validate our system, we compared HEK293 cells transiently transfected with a MultiLabel plasmid encoding five fluorescent proteins with cells co-transfected with individual parental expression vectors. Co-transfection led to an inhomogeneous mixture of cells, including many cells lacking expression of one or several proteins ( Fig. 2a ). In contrast, MultiLabel-transfected cells efficiently expressed all five fluorescent proteins at similar levels ( Fig. 2b ). Quantification of the expression levels at the single-cell level revealed a constant relationship between the expression levels of individual proteins ( Supplementary Fig. S7 ). 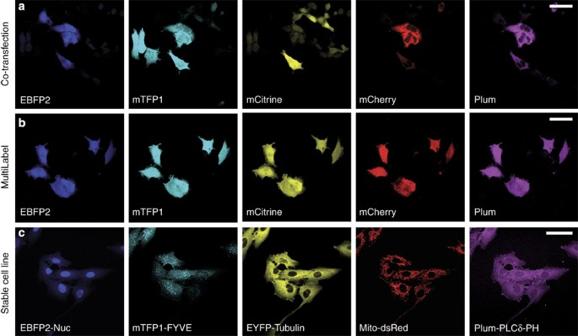Figure 2: Transient and stable modification of mammalian cells with MultiLabel. (a) HEK293 cells were transiently transfected with a mixture of five plasmids, each containing an expression cassette for a single fluorescent protein or (b) a single MultiLabel plasmid containing five expression cassettes for fluorescent proteins. See alsoSupplementary Figure S7for examples with 2, 3 and 4 expression cassettes, as well as quantification of expression levels. (c) Generation of stable cell lines. PAE cells were transfected with a linearized plasmid containing five expression cassettes for subcellular markers and then selected with G418. EBFP2-Nuc/EBFP2 with a nuclear localization signal; mTFP1-FYVE/mTFP1 with a PI-3-P binding FYVE domain; EYFP-Tubulin/EYFP fused to tubulin; Mito-dsRed/dsRed with mitochondrial localization; Plum-PLCδ-PH/Plum fused to the PI-4,5-P2 binding pleckstrin homology domain of PLCδ. Supplementary Movie 1 shows a time-lapse movie of this cell line. Scale bars, 50 μm. Figure 2: Transient and stable modification of mammalian cells with MultiLabel. ( a ) HEK293 cells were transiently transfected with a mixture of five plasmids, each containing an expression cassette for a single fluorescent protein or ( b ) a single MultiLabel plasmid containing five expression cassettes for fluorescent proteins. See also Supplementary Figure S7 for examples with 2, 3 and 4 expression cassettes, as well as quantification of expression levels. ( c ) Generation of stable cell lines. PAE cells were transfected with a linearized plasmid containing five expression cassettes for subcellular markers and then selected with G418. EBFP2-Nuc/EBFP2 with a nuclear localization signal; mTFP1-FYVE/mTFP1 with a PI-3-P binding FYVE domain; EYFP-Tubulin/EYFP fused to tubulin; Mito-dsRed/dsRed with mitochondrial localization; Plum-PLCδ-PH/Plum fused to the PI-4,5-P2 binding pleckstrin homology domain of PLCδ. Supplementary Movie 1 shows a time-lapse movie of this cell line. Scale bars, 50 μm. Full size image Generation of stable cell lines We have created acceptor plasmids that contain an Flp-In cassette for recombination-based integration into mammalian genomes and a G418 resistance gene to select for random integration (see Supplementary Fig. S3 ). The Flp-In system allows the recombination-based integration of a single copy of a transgene at a defined position [9] (distributed by Invitrogen). This system is therefore very useful to test a series of mutants in a cell biological assay. Efficient FRT-based integration into Flp-In cells occurred with circular MultiLabel constructs smaller than 15 kb. For integration of larger MultiLabel plasmids, we linearized the multigene construct by cleaving at a unique homing-endonuclease site (I-SceI in pSI-AKR7 and AAL6; Supplementary Fig. S3 ). Only the transfection of such linearized plasmids allowed the generation of cell lines simultaneously expressing several transgenes ( Fig. 2c ). Supplementary Movie 1 is a time-lapse movie of this cell line expressing five subcellular markers with fluorescent tags (EBFP2-Nuc, mTFP1-FYVE, EYFP-Tubulin, Mito-dsRed and Plum-PLCδ-PH). To maximize integration efficacy, we next created an acceptor vector (pSI-AKR8) with two eukaryotic selection markers. Digestion of an assembly based on pSI-AKR8 with I-SceI leads to a linear fragment with selection markers at both ends ( Supplementary Fig. S8 ). Only cells that integrate the entire fragment with all its expression cassettes and the flanking resistance markers will survive selection with G418 and zeocin. Biochemical analysis of transiently transfected cells The transfection efficiency of a 21 kb construct encoding five fluorescent proteins was approximately 20% in HEK293 cells and 1–5% in Porcine aortic endothelial or COS cells. The expression levels of 20–25 kb constructs encoding for instance receptor tyrosine kinases and associated proteins were sufficient for biochemical analysis. We were then interested in whether the expression ratios are identical for acceptor–donor1–donor2 and acceptor–donor2–donor1 constructs. We compared the relative expression levels of an SNX5–SNX1–EGFR (1.0/1.4/0.3) to an SNX5–EGFR–SNX1 (1.0/1.5/0.3) construct. Likewise, the comparison of SNX5–SNX2–EGFR (1.0/1.2/0.7) with SNX5–EGFR–SNX2 (1.0/1.2/0.8)-transfected cells showed similar expression ratios for all proteins ( Fig. 3 ). The sequence of the assembly is therefore not important for expression. 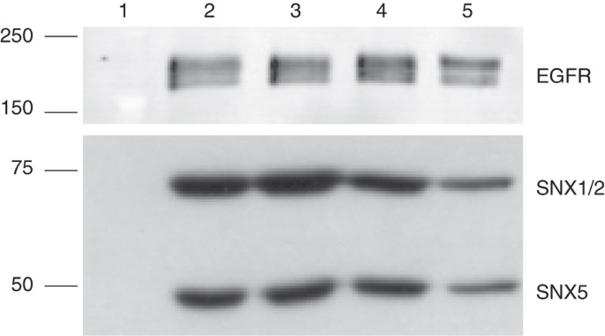Figure 3: Transient transfection of HEK293 cells with a MultiLabel plasmid. All constructs encode myc-SNX5 (acceptor in all four constructs), EGFR (Donor1) and myc-SNX1 or myc-SNX2 (donor2). The expression cassettes are arranged in the following sequence: SNX5–SNX1–EGFR (lane 2), SNX5–EGFR–SNX1 (lane 3), SNX5–SNX2–EGFR (lane 4) and SNX5–EGFR–SNX2 (lane 5). Lysates from untransfected cells were loaded on lane 1. The transfection efficiency is sufficient for biochemical analysis by western blotting. The different order of the expression cassette (SNX5–SNX1–EGFR versus SNX5–EGFR–SNX1) has no influence on relative expression levels. Molecular weights are shown in kDa. Figure 3: Transient transfection of HEK293 cells with a MultiLabel plasmid. All constructs encode myc-SNX5 (acceptor in all four constructs), EGFR (Donor1) and myc-SNX1 or myc-SNX2 (donor2). The expression cassettes are arranged in the following sequence: SNX5–SNX1–EGFR (lane 2), SNX5–EGFR–SNX1 (lane 3), SNX5–SNX2–EGFR (lane 4) and SNX5–EGFR–SNX2 (lane 5). Lysates from untransfected cells were loaded on lane 1. The transfection efficiency is sufficient for biochemical analysis by western blotting. The different order of the expression cassette (SNX5–SNX1–EGFR versus SNX5–EGFR–SNX1) has no influence on relative expression levels. Molecular weights are shown in kDa. Full size image Cells expressing multiple proteins show normal physiology Finally, we validated the MultiLabel system in a cell biological assay using a set of plasmids encoding fluorescently tagged sensors. The Rab sensors express the small GTPases Rab5, Rab4 and Rab11 or Rab5, Rab4 and Rab7. These proteins are associated with different vesicles in the endosomal compartment [10] . The phosphoinositide (PI) sensor recognizes PI-3-P (FYVE domain), PI-4,5-P2 (PLCδ-PH) and PI-3,4,5-P3 (BTK-PH) [11] . COS cells, which endogenously express the epidermal growth factor receptor (EGFR), were transiently transfected with these sensor constructs and then stimulated with fluorescently labelled EGF (EGF-Alexa647). Twenty minutes after stimulation of cells with EGF-Alexa647, the EGFR was co-localized with PI-3-P, Rab5 and Rab4, showing that the receptor was internalized as expected. Minor co-localization with Rab11 was observed (recycling endosomes). In addition, EGF-induced plasma membrane ruffles positive for PI-3,4,5-P3 were observed ( Fig. 4a,b ). 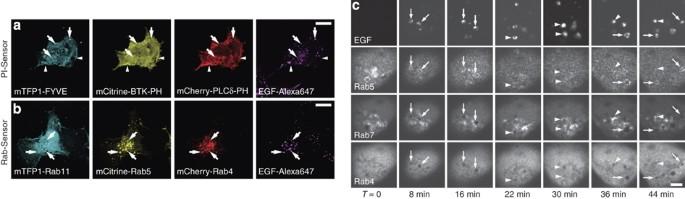Figure 4: Monitoring of the EGFR in activated COS cells. COS cells were transiently transfected with a construct encoding (a) three different phosphoinositide-binding proteins or (b) three different Rab proteins and then stimulated with EGF-Alexa647 for 20 min. At this time point, the EGFR co-localized with the PI-3-P-binding FYVE domain (arrows) in early endosomes. In addition, EGF-induced ruffles at the plasma membrane were positive for PI-3,4,5-P3 (BTK-PH) and PI-4,5-P2 (PLCδ-PH) (arrowheads). In cells expressing the Rab sensor, the EGFR co-localized mainly with Rab5 and Rab4 (arrows). (c) COS cells were transiently transfected with a MultiLabel plasmid encoding mCitrine-Rab5, mTFP1-Rab4 and mCherry-Rab7. Cells were stimulated with EGF-Alexa647 and monitored for 45 min. As expected, EGF was found in Rab5-positive vesicles shortly after addition (T=8/T=16, arrows). Later, it was also found in Rab7-positive vesicles (arrowheads). Scale bars, 50 μm (a,b); 5 μm (c). A time-lapse series of an EGF-stimulated COS cell transfected with mCitrine-Rab5, mCherry-Rab7 and mTFP1-Rab4 is shown in Figure 4c . The EGFR co-localized initially exclusively with Rab5 (early endosomes) and later with Rab5 and Rab7 (late endosomes). EGF was mainly found within vesicles, whereas Rab proteins were found on the membrane of vesicles. Very often, only subcompartments of vesicles were positive for Rab proteins. These results indicate that the normal physiology of cells was not disturbed when these sensors were simultaneously expressed. Figure 4: Monitoring of the EGFR in activated COS cells. COS cells were transiently transfected with a construct encoding ( a ) three different phosphoinositide-binding proteins or ( b ) three different Rab proteins and then stimulated with EGF-Alexa647 for 20 min. At this time point, the EGFR co-localized with the PI-3-P-binding FYVE domain (arrows) in early endosomes. In addition, EGF-induced ruffles at the plasma membrane were positive for PI-3,4,5-P3 (BTK-PH) and PI-4,5-P2 (PLCδ-PH) (arrowheads). In cells expressing the Rab sensor, the EGFR co-localized mainly with Rab5 and Rab4 (arrows). ( c ) COS cells were transiently transfected with a MultiLabel plasmid encoding mCitrine-Rab5, mTFP1-Rab4 and mCherry-Rab7. Cells were stimulated with EGF-Alexa647 and monitored for 45 min. As expected, EGF was found in Rab5-positive vesicles shortly after addition ( T =8/ T =16, arrows). Later, it was also found in Rab7-positive vesicles (arrowheads). Scale bars, 50 μm ( a , b ); 5 μm ( c ). Full size image Heterologous multigene expression in mammalian cells is a key technology in contemporary biological research. Unfortunately, all available technologies suffer from major deficiencies such as unreliable co-transfection efficiency. Our MultiLabel system is clearly superior to the currently available technology for a number of reasons. Several expression cassettes can be assembled in a combinatorial way because the system is modular. This is a clear advantage when combinations of proteins or mutations of a protein need to be tested. All cells express the entire set of transfected genes. Therefore, the population of transfected cells is uniform and not a mixture of cells expressing only a fraction of the transfected genes, a fact that is especially important in biochemical assays. Simultaneous insertion of several genes into a cell genome is possible in a single step, which is less time-consuming than sequential integration by multiple transfections. The expression levels can be regulated independently because the system transcribes autonomous mRNAs and is not polycistronic. The use of IRES elements often leads to unpredictable expression of the adjacent genes. Several cloning strategies, including robotics-based high-throughput methods, can be used because of the application of standardized cloning sites. The assembly of the expression cassettes is recombination based and therefore independent of restriction enzymes. Our design also allows the rapid modification of acceptor and donor vectors, thus extending the scope of our technology to viral expression or to different integration systems. Our results provide evidence for the first time that it is possible to use this technology concept to perform cell biological assays with high efficacy. Our results clearly demonstrate that the behaviour of the transfected cells is not negatively affected, that we can reproduce previously published intracellular trafficking studies and that the transfected cells are evidently still able to proliferate. Most contemporary time-lapse movies and time-course studies typically show only two colour channels. In contrast, we show here a time course of a transiently transfected cell with four channels and a movie of a cell line with five channels. Taken together, this provides compelling evidence that MultiLabel indeed addresses and alleviates hitherto inhibiting technical problems. We anticipate that a broad range of applications in cell biology will significantly benefit from the MultiLabel system. In this study, using fluorescent markers, we demonstrate the superior performance of MultiLabel when compared with conventional coexpression systems. By introducing affinity purification tags, our approach will be of equal benefit for systems and structural biology applications in mammalian cells. We considerably extend the existing tool box for expression of protein and protein complexes, for instance, in the context of applications in drug development and screening. Molecular biology PCR fragments were generated with Phusion DNA Polymerase (Finnzymes) or Taq Plus Precision (Stratagene). Primers and templates are depicted in Supplementary Table S1 and in Supplementary Methods . These fragments, including the regulatory elements, were cloned into the pGEM-T vector (Promega). Fragments were cut from these vectors with SapI (LguI), isolated from TAE agarose gels, purified with the Qiaquick gel extraction kit (Qiagen) and then stored at −20 °C. Donor and acceptor vectors were created in a single ligation step of eight fragments ( Supplementary Fig. S1 ). The consensus sequence and the nomenclature of these plasmids are given in Supplementary Figure S2 . The available donor and acceptor vectors are shown in Supplementary Figure S3 . Plasmids containing a pUC origin of replication were propagated in TopTen or DH10β cells, and plasmids with an R6Kγ origin of replication in pir + cells [6] . The genes of interest were cloned into donor and acceptor vectors with T4 DNA ligase or SLIC [12] . Note that existing expression vectors from the pcDNA (Invitrogen) or pEGFP (Clontech) type can be amplified with standard primers and inserted into the desired backbone ( Supplementary Fig. S4 ). The Cre/ LoxP recombination reaction was performed at 37 °C for 60 min (New England BioLabs). We recommend using plasmids that were purified with an anion exchange method. Three plasmids can be routinely assembled in a single step. The fourth or fifth plasmid can be inserted in a sequential manner and highly competent cells should be used. Note that there are two possibilities for assembling three plasmids, six possibilities for assembling four plasmids and 24 possibilities for assembling five plasmids. The unpurified Cre reaction mixture was used to transform DH10β or TopTen cells by electroporation. The transformation efficiency of fusions containing four or five plasmids was optimized by culturing the transformed cells overnight at 30 °C in liquid culture containing appropriate antibiotics before plating and/or by using highly competent commercial cells. Plasmids should be analysed by digestion with restriction enzymes. Antibiotics were used in the following concentrations for assemblies of 1–3 plasmids: ampicillin, 50 μg μl −1 ; kanamycin, 25 μg μl −1 ; spectinomycin, 50 μg μl −1 ; chloramphenicol, 4 μg μl −1 ; and gentamycin, 4 μg μl −1 . Antibiotic concentrations were reduced to 50% when four or five plasmids were assembled. Rearrangement or denaturation of plasmids during growth was eliminated by culturing the bacteria in Luria-Bertani (LB) medium at 30 °C rather than by using 2×YT at 37 °C. Cell culture HEK293 and COS cells were maintained at 37 °C with 5% CO 2 in DMEM (Amimed) containing 10% fetal calf serum (Amimed), 100 units ml −1 penicillin and 100 μg ml −1 streptomycin (Invitrogen). HAM-F12 (Amimed) was used instead of DMEM for Porcine aortic endothelial cells. Cells were transfected with Fugene HD (Roche) or with calcium phosphate. MultiLabel plasmids were diluted with carrier plasmids (1:3 or 1:5) when the expression level was too high. Stable cell lines were generated with the Flp-In system according to the manufacturer's recommendations (Invitrogen) or by random integration of linearized plasmids. Selection was performed with the following antibiotics and concentrations: G418, 16 μg ml −1 (Calbiochem); hygromycin, 50 μg ml −1 (Roche); zeocin, 100 μg μl −1 (Invitrogen). Homing endonucleases were obtained from New England Biolabs. Microscopy Cells were plated on glass coverslips, cultured for 40 h and then fixed with 4% formaldehyde (either directly in the culture medium or in PBS). Samples were washed three times with PBS and then mounted with Citifluor AF1. Imaging was performed on a Leica SP5 laser scanning confocal microscope or on an Olympus IX81 equipped with an Andor iXon EM camera ( Supplementary Movie 1 ). Emission windows of the fluorescent proteins were defined with a construct expressing five non-overlapping fluorescence-tagged subcellular markers. EBFP2 was excited with the 405 nm laser line and emission was collected from 430 to 450 nm (405/430–450). The other fluorescent proteins were analysed as follows: mTFP1 (458/485–510); mCitrine (514/525–545); mCherry (543/585–620); mPLUM (633/640–800). In addition, the spectral mode (xyλ) of the microscope was used to verify the presence of all fluorescent proteins (data not shown). Quantification was performed with LAS AF software (Leica Microsystems). Figures were processed with Photoshop or Imaris software (Bitplane). Gaussian filter, brightness and contrast including gamma adjustment were used to increase the visibility of vesicles. All operations were carried out on the entire set of images. Western blotting HEK293 cells were plated in 6 cm dishes at a density of 50% 1 day before transfection. Cells were transfected with FugeneHD according to the manufacturer's recommendations (Roche) and lysed 40 h later with lysis buffer (0.5% Triton X-100, 50 mM Tris–HCl, 100 mM NaCl). The supernatant was used for western blotting after sonification and centrifugation. Antibodies used were rabbit anti-EGFR (Neomarkers, RB-1417, diluted 1:1,000 in 3% BSA/TBST) and mouse anti-myc-tag (9E10, diluted 1:5 in 3% BSA/TBST). As secondary antibodies, alkaline phosphatase-coupled goat anti-mouse (Southern Biotech, 1031-04, diluted 1:10,000 in 3% milk powder/TBST) and anti-rabbit (Southern Biotech, 4050-04, diluted 1:10,000 in 3% milk powder/TBST) antibodies were used, followed by chemiluminescene detection. How to cite this article: Kriz, A. et al . A plasmid-based multigene expression system for mammalian cells. Nat. Commun. 1:120 doi: 10.1038/ncomms1120 (2010).